Bioreactor droplets from liposome-stabilized all-aqueous emulsions Artificial bioreactors are desirable for in vitro biochemical studies and as protocells. A key challenge is maintaining a favourable internal environment while allowing substrate entry and product departure. We show that semipermeable, size-controlled bioreactors with aqueous, macromolecularly crowded interiors can be assembled by liposome stabilization of an all-aqueous emulsion. Dextran-rich aqueous droplets are dispersed in a continuous polyethylene glycol (PEG)-rich aqueous phase, with coalescence inhibited by adsorbed ~130-nm diameter liposomes. Fluorescence recovery after photobleaching and dynamic light scattering data indicate that the liposomes, which are PEGylated and negatively charged, remain intact at the interface for extended time. Inter-droplet repulsion provides electrostatic stabilization of the emulsion, with droplet coalescence prevented even for submonolayer interfacial coatings. RNA and DNA can enter and exit aqueous droplets by diffusion, with final concentrations dictated by partitioning. The capacity to serve as microscale bioreactors is established by demonstrating a ribozyme cleavage reaction within the liposome-coated droplets. Artificial microreactors are appealing as a way to gain insight into biological compartmentalization and for applications in biotechnology and medicine. At its most basic, a microreactor consists of a semipermeable shell through which reactants and products can pass and an interior environment where reactions can occur. Notable examples of compartments that have been used as microreactors include liposomes [1] , polymer capsules [2] , [3] , colloidosomes [4] , [5] , hydrogels and liquid–liquid emulsions (oil/water [6] , [7] , aqueous/aqueous [8] , [9] , [10] ), in which individual droplets can be considered as microreactors [11] . Interior reactivity can be facilitated by catalysts that are either physically trapped in the interior (for example, by a membrane), or concentrated there on the basis of preferential solubility (for example, in a water/oil biphasic system) [6] . A key challenge for the design of artificial bioreactors is maintaining reaction-relevant internal environments (for example, containing catalysts, macromolecular crowders) while allowing entry/egress of substrates and products. Here, we introduce liposome-stabilized all-aqueous emulsion droplets as a new class of bioreactors that simultaneously achieve these goals. The internal microenvironment is a distinct phase composition into which solutes can be selectively concentrated, and the semipermeable shell is composed of intact ~130-nm diameter liposomes, between which solutes may pass to enter or exit the microscale bioreactors. Aqueous two-phase systems (ATPS), such as the well-known PEG/dextran system [12] , are attractive as biomimetic media because they offer coexisting macromolecularly crowded aqueous compartments with different chemical and physical properties separated by a low-energy boundary, across which solutes such as proteins or nucleic acids can equilibrate without denaturation [10] , [13] , [14] . This is similar to biological fluids such as the cytoplasm and nucleoplasm, which contain 17–40 wt% biomacromolecules [15] , [16] . Crowding can considerably alter kinetics and thermodynamics for many biochemical reactions [17] , for example PEG and dextran polymers favour reactivity of the CPEB3 ribozyme [18] . In the PEG/dextran system, RNA partitions strongly to the dextran-rich phase [10] , [12] . This effect, which is length-dependent, has been used to increase ribozyme reaction rates up to nearly 70-fold by localization in the dextran-rich phase [10] . Recent studies suggest that aqueous phase separation is responsible for some forms of microcompartmentalization in vivo [19] . Partitioning of solutes such as proteins, nucleic acids or small molecules into aqueous phase compartments provides a mechanism for microcompartmentalization and localized reactivity. Unlike intracellular compartments that can persist at the micron scale indefinitely, a typical ATPS requires mechanical agitation to maintain microscale droplets, as coalescence into macroscale phases occurs in quiescent samples. For water-in-oil systems, emulsification is routinely accomplished using amphiphilic surfactants that adsorb at the water/oil interface. This approach, while not impossible for ATPS [20] , [21] , is much more challenging due to the chemical similarity of the two aqueous media. An alternative means of stabilizing a liquid/liquid interface is adsorption of particles to form a Pickering emulsion [22] . In a typical Pickering emulsion, micron-scale polystyrene or silica particles adsorb at an oil–water interface, where they can provide a steric barrier against droplet coalescence [23] . The driving force for particle adsorption (Δ E ) depends on particle radius ( R ), interfacial tension ( γ) , and contact angle ( θ ), with Δ E =−π R 2 γ (1−|cos θ |) 2 (ref. 24 ). Although ATPS have low interfacial tensions relative to oil/water systems [12] , [25] , cells, liposomes and microparticles have been observed at the aqueous/aqueous interface of bulk ATPS [26] , [27] , [28] , [29] , [30] , [31] , [32] , [33] , [34] , [35] . Recently, formation of water-in-water phase systems stabilized by latex beads [27] , fat globules [28] or protein particles have been reported [29] . It is not unreasonable to anticipate that intracellular liquid/liquid interfaces would similarly accumulate particulates [14] . Here, we demonstrate Pickering-type emulsions upon assembly of negatively charged, ~130-nm diameter liposomes at the aqueous/aqueous interface of a PEG/dextran ATPS. The resulting liposome-coated, polymer-rich aqueous phase droplets are shown to serve as microreactors that confine a ribozyme while permitting substrate and product transport. These structures can be thought of as a primitive model cell or protocell [36] , [37] , [38] , in which partitioning both simplifies ‘loading’ with polymeric crowding agents and bioactive molecules such as RNA, and indefinitely maintains distinct internal and external solute concentrations, while the liposomal coating prevents coalescence without sealing off the internal volume from solute entry or egress. Formation of liposome-stabilized all-aqueous emulsions When PEGylated liposomes [39] (for synthesis and analysis, see Supplementary Methods), ~130 nm in diameter and consisting primarily of egg phosphatidyl glycerol (PG), are mixed with a PEG/dextran ATPS, an emulsion is formed in which microscale droplets of one phase, surrounded by a liposome layer, are suspended in the other phase. Droplet coalescence is strongly inhibited as determined by turbidity measurements, though droplets sediment or rise (cream) over many hours due to phase density differences ( Supplementary Fig. 1 ). Inspection using confocal fluorescence microscopy shows labelled lipid at the aqueous/aqueous interface surrounding micron-scale droplets of the dispersed phase ( Fig. 1 ). The identity of the continuous and dispersed phases can be controlled by altering their relative volumes. Emulsions form when the continuous phase is PEG-rich, with the dispersed phase dextran-rich, as well as when the phases are inverted ( Fig. 1 ). Stable inverted emulsions are not expected for a stabilized emulsion of this particle size from sterics alone [40] . For small particles to form a large enough steric barrier to stabilize, they must favour the continuous phase (particle-droplet contact angle <90°). When the emulsion is inverted, these particles favour what is now the dispersed phase and consequently cannot form an effective steric barrier. Although our liposomes are too small to enable direct determination of contact angle, their ability to stabilize droplets of either phase suspended in the other argues against a steric stabilization mechanism for this system. 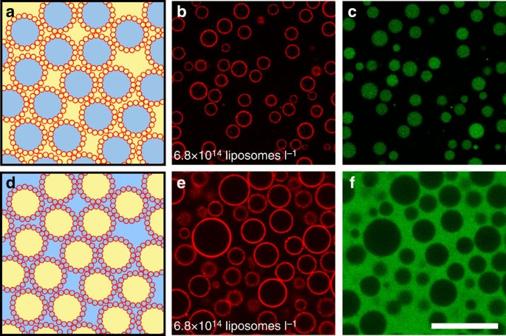Figure 1: Liposome-stabilized ATPS emulsions. (a,b, andc) Dextran-rich droplets dispersed in PEG-rich continuous phase. (a) Schematic illustration (red, liposomes; blue, dextran-rich phase; and yellow, PEG-rich phase), (b) fluorescence image showing location of DOPE-Rhodamine-labelled liposomes at the aqueous/aqueous interface, (c) fluorescence image showing location of dextran-rich phase labelled with fluorescein isothiocyanate (FITC)-dextran 500 kDa. The inverted emulsion is depicted as (d) an illustration, (e) a fluorescence image showing location of DOPE-Rhodamine-labelled liposomes at the aqueous/aqueous interface, (f) a fluorescence image showing location of dextran-rich phase labeled with FITC-dextran 500 kDa. Liposome concentrations were 6.8 × 1014liposomes l−1. All image frames use the 25 μm scale bar. Figure 1: Liposome-stabilized ATPS emulsions. ( a , b , and c ) Dextran-rich droplets dispersed in PEG-rich continuous phase. ( a ) Schematic illustration (red, liposomes; blue, dextran-rich phase; and yellow, PEG-rich phase), ( b ) fluorescence image showing location of DOPE-Rhodamine-labelled liposomes at the aqueous/aqueous interface, ( c ) fluorescence image showing location of dextran-rich phase labelled with fluorescein isothiocyanate (FITC)-dextran 500 kDa. The inverted emulsion is depicted as ( d ) an illustration, ( e ) a fluorescence image showing location of DOPE-Rhodamine-labelled liposomes at the aqueous/aqueous interface, ( f ) a fluorescence image showing location of dextran-rich phase labeled with FITC-dextran 500 kDa. Liposome concentrations were 6.8 × 10 14 liposomes l −1 . All image frames use the 25 μm scale bar. Full size image To learn more about the stabilization mechanism for these emulsions, we measured the average droplet size as a function of liposome concentration. Droplet size for a constant ATPS composition was inversely correlated with liposome concentration ( Fig. 2a ). Smaller droplets were observed as more liposomes were added, consistent with strong liposome adsorption at the interface. At higher liposome concentrations, droplet size levels off. A similar trend has been reported for nanoparticle-stabilized oil/water Pickering emulsions, which form close-packed monolayers [24] . Based on our observed droplet size, liposome size and geometry; liposome coverage at the interface can be estimated. As shown in Fig. 2b , an approximation (see Supplementary Note 1 and Supplementary Equations (1–8) ) based on two layers of close-packed liposomes predicts consistently larger droplet sizes than observed, indicating that liposome multilayers are not forming at the aqueous/aqueous interface. An estimation for monolayer packing is closer to the experimental data, but the closest match to our data is a submonolayer of liposomes, suggesting that there is unoccupied interface between the liposomes at concentrations <0.4 × 10 16 liposomes l −1 ( Fig. 2b ). 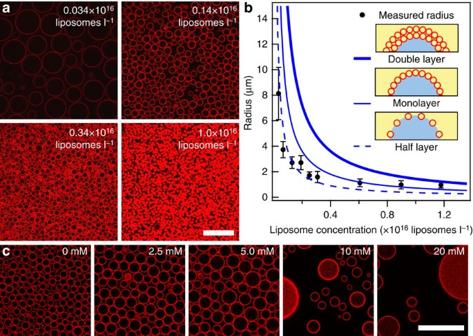Figure 2: Droplet size in the emulsion depends on lipsome concentration and solution ionic strength. All images are of Rhodamine-labelled liposomes and are of dextran-rich droplets in PEG-rich continuous phase. (a) Microscopy images show that the size of droplets is inversely correlated with the concentration of liposomes. Scale bar, 25 μm. (b) The size of droplets is liposome concentration dependent. The blue lines represent droplet sizes predicted from assuming different numbers of hexagonally close-packed lipsomes in varying numbers of planar layers, and the inset shows the different possibilities of packing. For each concentration,n=450 droplets were counted and error bars represent standard deviations. (c) Screening of charge leads to emulsion destabilization (concentration=1.4 × 1015liposomes l−1). At low ionic strength, a reduction in Debye length leads to tighter liposome packing at the interface, increasing the observed droplet size (2.5 and 5 mM added NaCl). As ionic strength increases, the liposomes can no longer prevent droplet coalescence. Scale bar, 25 μm. Figure 2: Droplet size in the emulsion depends on lipsome concentration and solution ionic strength. All images are of Rhodamine-labelled liposomes and are of dextran-rich droplets in PEG-rich continuous phase. ( a ) Microscopy images show that the size of droplets is inversely correlated with the concentration of liposomes. Scale bar, 25 μm. ( b ) The size of droplets is liposome concentration dependent. The blue lines represent droplet sizes predicted from assuming different numbers of hexagonally close-packed lipsomes in varying numbers of planar layers, and the inset shows the different possibilities of packing. For each concentration, n =450 droplets were counted and error bars represent standard deviations. ( c ) Screening of charge leads to emulsion destabilization (concentration=1.4 × 10 15 liposomes l −1 ). At low ionic strength, a reduction in Debye length leads to tighter liposome packing at the interface, increasing the observed droplet size (2.5 and 5 mM added NaCl). As ionic strength increases, the liposomes can no longer prevent droplet coalescence. Scale bar, 25 μm. Full size image Stabilization against droplet coalescence at submonolayer liposome coverage is consistent with charge repulsion due to the negative charges on the liposomes and the low ionic strength at which these experiments were performed (Debye screening length, κ −1 , ~25 nm). We note that in oil–water Pickering emulsions large differences in electric permittivity between the phases results in large differences in ion concentrations between phases and leads to complex electrostatic effects [40] , [41] , [42] , [43] . In contrast, much smaller differences in permittivity exist between the PEG-rich and dextran aqueous phases used here, and concentrations of small ions (for example, Na + ) are the same in both phases. Electrostatic repulsion increases the effective interfacial area occupied by each liposome. We therefore suggest an electrostatic stabilization mechanism for these liposome-stabilized, all-aqueous emulsions. Indeed, when charges are screened, reduced liposome spacing yields increased droplet size and fluorescence intensity at the interface, as less interfacial area can be stabilized ( Fig. 2c , 2.5–5 mM NaCl). At 10 mM NaCl (κ −1 =3 nm), droplet coalescence was observed as electrostatic repulsion no longer prevented inter-droplet contact. Nature of the interfacial layer We proceeded to test whether the lipid vesicles remain intact after collecting at the aqueous/aqueous interface, rather than aggregating or fusing to form larger liposomes, bilayers or other structures. Fluorescence recovery after photobleaching experiments show essentially no recovery of lipid fluorescence, suggesting that interface-assembled lipid-containing structures are relatively immobile rather than diffusing either as individual lipids within bilayers or as interfacially bound liposomes ( Fig. 3a ). To determine if the absence of diffusion indicates liposome aggregation, we diluted the ATPS with an isotonic fructose solution to remove the aqueous/aqueous boundary and release the assembled material ( Supplementary Fig. 2 ). Dynamic light scattering was used to determine the size of lipid structures in the resulting single-phase solution. Even after 24 h at the interface, diameters for released liposomes were unchanged, indicating that liposomes remained intact rather than aggregating or fusing ( Supplementary Fig. 3 ). Arrested in-plane diffusion of microparticles has been observed for Pickering emulsions under ‘jamming’ conditions, where particle coverages at the interface are so high that individual particles cannot move [44] . Based on estimations of total stabilized surface area and liposome concentrations ( Fig. 2b ), we expect that the apparent jamming in our system is due to longer-range electrostatic repulsions between the negatively charged liposomes at the interface when ionic strength is low, but may be steric when charges are screened. 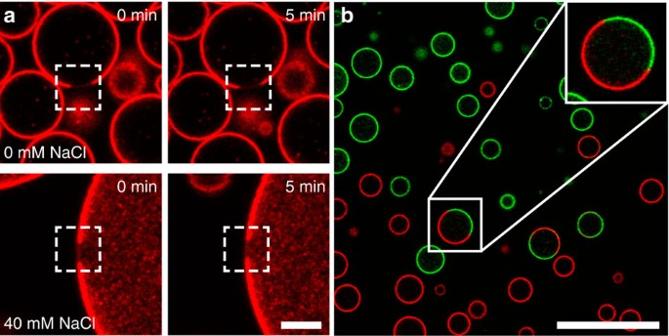Figure 3: Interfacial liposomes and partitioning solutes have different mobility. (a) Fluorescence recovery after photobleaching experiments show no recovery for PEGylated egg PG liposomes at the interface at both 0 and 40 mM NaCl. The bleached area in both 0 and 40 mM NaCl samples show no recovery after 5 min for particles’ diffusion to be this slow, jamming must be present. In the 0 mM NaCl case, the jamming is most likely electrostatic, whereas the 40 mM samples would exhibit steric jamming. The difference in mechanism is suspected due to the change in Debye length, from ~25 to 1.5 nm; and because osmotic deflation should make the liposomes less spherical. (b) When droplets undergo ionic strength-induced coalescence, interfacial mobility of individual liposomes is low. Coalescence of separate populations prepared with NBD (green) and Rhodamine (red) liposomes show persistence of distinct green and red regions. The scale bar inais 4 μm, and the scale bar inbis 25 μm. Figure 3: Interfacial liposomes and partitioning solutes have different mobility. ( a ) Fluorescence recovery after photobleaching experiments show no recovery for PEGylated egg PG liposomes at the interface at both 0 and 40 mM NaCl. The bleached area in both 0 and 40 mM NaCl samples show no recovery after 5 min for particles’ diffusion to be this slow, jamming must be present. In the 0 mM NaCl case, the jamming is most likely electrostatic, whereas the 40 mM samples would exhibit steric jamming. The difference in mechanism is suspected due to the change in Debye length, from ~25 to 1.5 nm; and because osmotic deflation should make the liposomes less spherical. ( b ) When droplets undergo ionic strength-induced coalescence, interfacial mobility of individual liposomes is low. Coalescence of separate populations prepared with NBD (green) and Rhodamine (red) liposomes show persistence of distinct green and red regions. The scale bar in a is 4 μm, and the scale bar in b is 25 μm. Full size image We took advantage of the lack of in-plane liposome diffusion to form more complex, Janus-like droplets in which different liposomes coated different portions of the droplet. Here, emulsions prepared with nitrobenzoxadiazole (NBD)-labelled (green) liposomes were gently combined on a microscope slide with separately prepared emulsions having Rhodamine-labelled (red) liposomes under conditions of reduced stability to facilitate droplet coalescence (that is, 20 mM NaCl). Figure 3b was acquired 30 min after mixing, and shows the results of droplet coalescence—red and green liposomes have not mixed across the interface; but instead have remained in separate regions after the coalescence events, such that the appearance of each droplet suggests its coalescence history. In contrast to quiescent solutions, when two distinct emulsions are vigorously mixed the resulting population is intermediate in droplet size and in partitioned solute concentration after as little as 30 s, indicating that the liposome layers and dextran-rich droplets are disrupted during vortexing and reform as one uniform population ( Supplementary Fig. 4 ). Transport in/out of droplets We anticipated that the submonolayer coverage of our liposome-stabilized aqueous/aqueous interface might permit transport into and out of droplets despite the poor lateral mobility within the layers themselves. Indeed, even close-packed monolayers of spherical particles can provide routes for possible solute entry/egress through interstitial spaces [5] . We evaluated three different fluorescently tagged solutes for their ability to enter liposome-stabilized droplets in the absence of mechanical agitation: 20- and 43-nt single-stranded DNA oligonucleotides and unPEGylated liposomes. Each of the test solutes is negatively charged, providing electrostatic repulsion from the negatively charged liposome layer stabilizing the interface, although each had a partitioning preference for the dextran-rich phase that provided a driving force for entry and accumulation in the droplets. Without PEG in the membrane, ~130-nm diameter PG liposomes partition to the dextran-rich phase ( Supplementary Fig. 5 left). Partitioning changes from the dextran-rich phase to the interface as more PEGylated lipid is added to the membrane ( Supplementary Fig. 6 ) When unPEGylated (NBD-labelled, green) liposomes were added to the PEG-rich phase of the stabilized emulsion and vortexed to mix, subsequent imaging showed them strongly and uniformly partitioned into the dextran-rich phase rather than assembling at the interface, which was coated with PEGylated (red) liposomes ( Supplementary Fig. 5 centre). This is unsurprising since experiments described above indicated that emulsion droplets undergo reorganization upon mechanical mixing. However, when the unPEGylated (green) PG liposomes were added to liposome-stabilized ATPS emulsions in the PEG-rich phase without disrupting the layer of PEGylated (red) liposomes around the droplets, they were unable to enter the dextran-rich phase. Droplet interiors remained dark even after several hours ( Supplementary Fig. 5 right); the interfacial liposome layer provided a barrier to the entry of these ~130-nm diameter objects. When a similar experiment was conducted using labelled DNA oligonucleotides as smaller test solutes (hydrodynamic radii 4 nm (refs 45 , 46 )), we observed rapid uptake of the labelled DNA from the PEG-rich phase into the liposome-stabilized droplets, as well as slower DNA relocation between droplets ( Fig. 4 and Supplementary Fig. 7 ). In Fig. 4 , dye-labelled 20-nt DNA initially present in PEG-rich phase was added on the right-hand side into a liposome-stabilized emulsion without DNA on the left-hand side. When the two emulsions are initially connected, DNA (blue, top panels) becomes concentrated almost immediately into the liposome-coated dextran-rich droplets on the right-hand side (red, lower panels), where mixing of the continuous phases occurs and DNA is accessible in the region immediately around individual droplets. At the first time point (<30 s), droplets on the edge of the sample already contained substantial concentrations of the fluorescently labelled DNA, consistent with rapid nucleic acid diffusion in PEG/dextran ATPS [47] and suggesting that the liposome layer posed essentially no barrier to entry. Migration of the DNA across the field of droplets, however, was much slower; note the absence of DNA fluorescence (blue, top panels) on the left-hand side even after 30 min. DNA partitions strongly into the dextran-rich phase of this ATPS [10] , so once it enters it is largely retained. Lower DNA concentration in the continuous phase limits uptake in droplets away from the site of mixing. Transfer between adjacent droplets was strongly dependent on DNA length, with the longer oligonucleotide exhibiting much slower migration of labelled DNA across the field of droplets ( Supplementary Fig. 7 ). This observation, along with similar extent of diffusion at the first time point, is consistent with the length dependence of nucleic acid partitioning wherein longer oligonucleotides strongly favour the dextran-rich phase [10] . The accumulation of oligonucleotides from the continuous exterior phase generates a biofunctional microenvironment within the stabilized, macromolecularly crowded aqueous droplets. This suggests possible application of these all-aqueous emulsions as microscale bioreactors where local concentrations of catalytic and crowding agents are maintained not by physical entrapment, but by preferential partitioning. 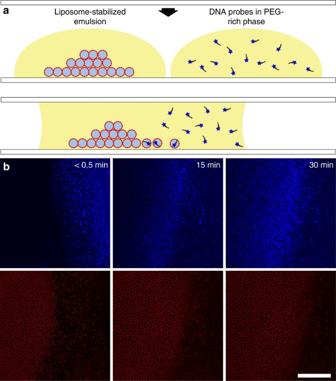Figure 4: Partitioning solutes can enter and exit the droplet through liposome-clad interface. (a) This cartoon depicts the two drops as they were arranged on the microscope coverslip, and how the top coverslip was used to bring them together. (b) Diffusion was observed at the edge of a collection of sedimented droplets after 20 nt DNA in a drop of PEG-rich phase was introduced by combining it with a drop of ATPS emulsion. Top and bottom panels show fluorescence channels for Alexa-647-labelled DNA (top) and Rhodamine-labelled liposomes that indicate the location of the droplets (bottom). For droplets near the edge, which were surrounded by the DNA containing PEG-rich phase upon mixing, fluorescence intensity corresponding to DNA accumulation inside was immediate (<30 s). Away from the site of initial mixing, the DNA concentration in the PEG-rich phase is lower; here, the intensity of labelled DNA inside droplets increases much more slowly as they equilibrate with neighbouring droplets. Droplets in this experiment were formed with 3 × 1014liposomes l−1. Scale bar, 500 μm. Figure 4: Partitioning solutes can enter and exit the droplet through liposome-clad interface. ( a ) This cartoon depicts the two drops as they were arranged on the microscope coverslip, and how the top coverslip was used to bring them together. ( b ) Diffusion was observed at the edge of a collection of sedimented droplets after 20 nt DNA in a drop of PEG-rich phase was introduced by combining it with a drop of ATPS emulsion. Top and bottom panels show fluorescence channels for Alexa-647-labelled DNA (top) and Rhodamine-labelled liposomes that indicate the location of the droplets (bottom). For droplets near the edge, which were surrounded by the DNA containing PEG-rich phase upon mixing, fluorescence intensity corresponding to DNA accumulation inside was immediate (<30 s). Away from the site of initial mixing, the DNA concentration in the PEG-rich phase is lower; here, the intensity of labelled DNA inside droplets increases much more slowly as they equilibrate with neighbouring droplets. Droplets in this experiment were formed with 3 × 10 14 liposomes l −1 . Scale bar, 500 μm. Full size image All-aqueous emulsion droplets as microscale bioreactors We tested the ability of the above structures to serve as bioreactors by performing a ribozyme cleavage reaction using a two-piece hammerhead ribozyme. 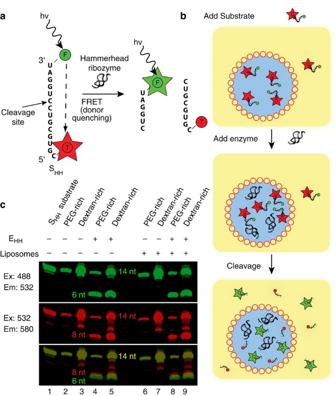Figure 5: Ribozyme cleavage reaction of a FRET-labelled substrate in an ATPS was evaluated by PAGE. (a) Fluorescent RNA substrate contains a donor that is quenched by FRET before cleavage and gains intensity after cleavage. (b) Substrate cleavage (second arrow) occurs in the microreactor following the addition of RNA enzyme strand (first arrow). Cleaved RNA products partition into the PEG-rich phase more than the larger substrate. The reaction was run in 2 mM MgCl2, 4 mM EDDS and 10 mM Tris pH 7.5 (seeSupplementary Fig. 8for importance of intermediate chelation by EDDS) (c) Gels show the reaction progress with and without liposomes, with controls to observe any substrate degradation in the absence of enzyme. SHHsubstrate is substrate HH, starting material in buffer alone. Data are after 1 h of reaction. Figure 5a,b illustrate the experimental design, in which a 43-nt enzyme strand binds to and cleaves a 14-nt substrate strand into 6- and 8-nt products ( Supplementary Table 1 ). This ribozyme is effectively confined within the bioreactor droplets with partitioning coefficient K =0.0063±0.0002, indicating ~ × 160 higher equilibrium concentration in the dextran-rich droplets as compared with the PEG-rich continuous phase. To monitor the reaction, the substrate strand was labelled with a pair of fluorescent dyes that exhibit Förster resonance energy transfer due to their proximity [48] , [49] . Upon cleavage of the substrate strand by the enzyme strand, the two dyes separate and donor fluorescence increases. In these reactions, changes were made to protect the liposomes from aggregation by Mg 2+ ions, which facilitate RNA enzyme activity. Liposomes were formed with 50:50 egg phosphatidylcholine and egg PG and an intermediate chelator, ethylenediamine disuccinic acid (EDDS), was added at 4 mM to protect the liposomes from aggregation by Mg 2+ ions. This chelator was determined experimentally to preserve liposome stability at 2 mM Mg 2+ so that stable droplets could be formed ( Supplementary Fig. 8 ). Figure 5: Ribozyme cleavage reaction of a FRET-labelled substrate in an ATPS was evaluated by PAGE. ( a ) Fluorescent RNA substrate contains a donor that is quenched by FRET before cleavage and gains intensity after cleavage. ( b ) Substrate cleavage (second arrow) occurs in the microreactor following the addition of RNA enzyme strand (first arrow). Cleaved RNA products partition into the PEG-rich phase more than the larger substrate. The reaction was run in 2 mM MgCl 2 , 4 mM EDDS and 10 mM Tris pH 7.5 (see Supplementary Fig. 8 for importance of intermediate chelation by EDDS) ( c ) Gels show the reaction progress with and without liposomes, with controls to observe any substrate degradation in the absence of enzyme. S HH substrate is substrate HH, starting material in buffer alone. Data are after 1 h of reaction. Full size image Both polyacrylamide gel electrophoresis and confocal fluorescence microscopy were employed to monitor the cleavage reaction ( Figs 5 and 6 , respectively). Polyacrylamide gel electrophoresis fractionation of isolated PEG-rich and dextran-rich phases yielded both reaction progress and partitioning data, while microscopy allowed us to visualize the reaction in real time. In Fig. 5c , lane 1 of the gel depicts the full-length substrate starting material in the absence of enzyme, and shows minimal substrate degradation over the course of the reaction. Lanes 2 and 3 show the ~1:2 partitioning of uncleaved substrate between the PEG-rich and dextran-rich phases, and lanes 6 and 7 show a similar partitioning trend in the presence of liposomes. The fluorescent substrate and product both favour the dextran-rich phase, although the partitioning to the dextran-rich phase is considerably less than for unmodified oligonucleotides of the same length ( Supplementary Table 1 ). We attribute this difference to the fluorescent labels, which contain large aromatic groups [12] . When the enzyme is added, the reaction proceeds. Apparent fractions cleaved are insensitive to the presence of liposomes, but are higher in the PEG-rich phase than the dextran-rich phase owing to the length dependence of oligonucleotide partitioning ( Fig. 5c , compare lanes 4 and 5, and 8 and 9; Supplementary Table 2 ). 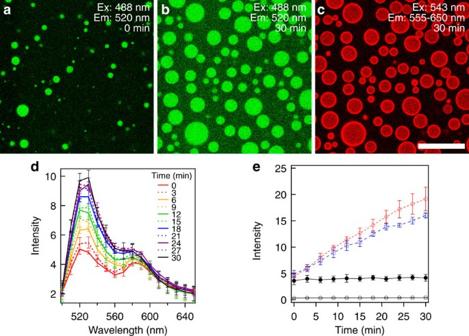Figure 6: The liposome-stabilized ATPS emulsion can be used as an RNA cleavage microreactor. (a,b) Fluorescein channel images showing increase in donor intensity in the PEG-rich phase over the course of the reaction. An increase in dextran-rich droplet number in the field of view is due to sedimentation. (c) The Rhodamine channel shows both acceptor fluorescence (imaged separately via FRET inSupplementary Figs 9–11) and the liposome tags. Liposomes appear as the bright ring surrounding the dextran-rich droplets. (d) Fluorescence emission spectra (Ex: 488 nm) in the PEG-rich phase are plotted during the reaction. The change comes both from a decrease in quenching and an increase in concentration due to repartitioning. (e) Reaction progress monitored in the PEG-rich phase. The values are calculated by subtracting the background to eliminate drift, and summing data from 520 and 530 nm to capture the donor peak (see Supplementary Methods). Plotted is the donor increase in the PEG-rich phase with liposomes (blue trace) and without liposomes (red trace), and degradation in the absence of enzyme (black line). Images for the controls without enzyme and without liposomes are found inSupplementary Figs 10 and 11. Scale bar, 25 μm. Figure 6: The liposome-stabilized ATPS emulsion can be used as an RNA cleavage microreactor. ( a , b ) Fluorescein channel images showing increase in donor intensity in the PEG-rich phase over the course of the reaction. An increase in dextran-rich droplet number in the field of view is due to sedimentation. ( c ) The Rhodamine channel shows both acceptor fluorescence (imaged separately via FRET in Supplementary Figs 9–11 ) and the liposome tags. Liposomes appear as the bright ring surrounding the dextran-rich droplets. ( d ) Fluorescence emission spectra (Ex: 488 nm) in the PEG-rich phase are plotted during the reaction. The change comes both from a decrease in quenching and an increase in concentration due to repartitioning. ( e ) Reaction progress monitored in the PEG-rich phase. The values are calculated by subtracting the background to eliminate drift, and summing data from 520 and 530 nm to capture the donor peak (see Supplementary Methods). Plotted is the donor increase in the PEG-rich phase with liposomes (blue trace) and without liposomes (red trace), and degradation in the absence of enzyme (black line). Images for the controls without enzyme and without liposomes are found in Supplementary Figs 10 and 11 . Scale bar, 25 μm. Full size image Confocal microscopy and microspectroscopy allowed visualization of individual droplet bioreactors. As the reaction proceeded, an increase in donor fluorescence was apparent in the PEG-rich continuous phase (compare Fig. 6a,b ), consistent with both loss of Förster resonance energy transfer and repartitioning of the donor-labelled product strands into the PEG-rich phase after enzymatic cleavage within the droplets. Indeed, the carboxyfluorescein (FAM)-labelled 6-nt product strand has reduced dextran-rich partitioning relative to the full-length substrate ( Supplementary Table 1 ). Reaction progress can be monitored by the increase in the donor emission (515–535 nm) from the PEG-rich phase ( Fig. 6d ), and is nearly the same with and without liposomes ( Fig. 6e ). Confocal microscopy data also confirmed that liposomes remained at the interface during the reaction ( Fig. 6c ). Hence, RNA catalysis is uninhibited by the liposome coating on the droplets, which as shown above stabilize the emulsion and provide some permselectivity. These data demonstrate feasibility of compartments that possess both a porous interface formed from the assembled liposomes and a macromolecularly crowded internal microenvironment that is chemically distinct from the external phase to serve as microscale bioreactors. Strong partitioning of the ribozyme, coupled with weaker partitioning for the substrate and almost no phase preference for the products helps to localize the reaction within the droplets and drive it towards completion by Le Chatelier’s principle as products re-equilibrate. Submicrometer diameter liposomes have been shown herein to stabilize all-aqueous emulsions against droplet coalescence. The liposomes partition strongly to the aqueous/aqueous interface, where they maintain their structure and are relatively immobile due to electrostatic jamming. This layer of negatively charged liposomes prevents droplet coalescence by electrostatic repulsion. These structures provide favourable microenvironments that support accumulation and reactivity of biomacromolecules as demonstrated with a ribozyme and can function as bioreactors. The submonolayer of individual PEGylated liposomes stabilizing the aqueous/aqueous interface offers a biocompatible interface that provides some degree of permselectivity by rejecting >100 nm liposomes but allowing 43-nt nucleic acids to pass through largely unimpeded. Although the charge stabilization mechanism observed here poses some limits on reaction conditions (that is, ionic strength) for which the emulsion is stable, this has been overcome here by use of intermediate chelation and we anticipate that additional stabilization methods, for example, use of larger lipid assemblies that offer greater steric stabilization, can be employed to expand applicable conditions. It is interesting to compare the assemblies observed here for liposomes at a PEG/dextran ATPS with those recently reported for fatty acid multilayers accumulating around coacervate droplets [50] . It appears that the assembly mechanism and observed structures are quite different between the fatty acid/coacervate and liposome/ATPS systems, indicating multiple routes to protocells and/or bioreactors in which polymer-rich liquid phases could become encapsulated within a semipermeable coating. In comparison with traditional giant liposomes, which encapsulate a similar aqueous volume in a uniform lipid bilayer membrane, the structures introduced here offer (1) facile encapsulation of macromolecular crowding agents and biomacromolecules by partitioning into the interior phase, (2) excellent uniformity in droplet size and contents across a population, (3) much greater access into/out of the interior volume. This could offer substantial advantages in bioreactor construction, particularly for biomimetic systems where complex mixtures of macromolecules in nearly identical interior microenvironments are desirable across a population of bioreactors, and where the impermeability of giant vesicle lipid bilayer membranes to even relatively small solutes restricts the types of reactions that can be performed. The observation that aqueous/aqueous interfaces can template assembly of liposome submonolayers also suggests the intriguing possibility that such structures could ultimately be converted into contiguous lipid bilayer membranes by rupture and in-plane restructuring of the assembled liposomes, similar to the formation of supported lipid bilayers on bare and polymer-coated solid surfaces [51] , [52] , [53] . Such a process would be of interest for generating uniform populations of ‘pre-loaded’ artificial cells and could serve as a mechanism for cellularization of primitive Pickering-style protocells. How to cite this article: Dewey, D. C. et al . Bioreactor droplets from liposome-stabilized all-aqueous emulsions. Nat. Commun. 5:4670 doi: 10.1038/ncomms5670 (2014).